CSN6 drives carcinogenesis by positively regulating Myc stability Cullin-RING ubiquitin ligases (CRLs) are critical in ubiquitinating Myc, while COP9 signalosome (CSN) controls neddylation of Cullin in CRL. The mechanistic link between Cullin neddylation and Myc ubiquitination/degradation is unclear. Here we show that Myc is a target of the CSN subunit 6 (CSN6)–Cullin signalling axis and that CSN6 is a positive regulator of Myc. CSN6 enhanced neddylation of Cullin-1 and facilitated autoubiquitination/degradation of Fbxw7, a component of CRL involved in Myc ubiquitination, thereby stabilizing Myc. Csn6 haplo-insufficiency decreased Cullin-1 neddylation but increased Fbxw7 stability to compromise Myc stability and activity in an Eμ-Myc mouse model, resulting in decelerated lymphomagenesis. We found that CSN6 overexpression, which leads to aberrant expression of Myc target genes, is frequent in human cancers. Together, these results define a mechanism for the regulation of Myc stability through the CSN–Cullin–Fbxw7 axis and provide insights into the correlation of CSN6 overexpression with Myc stabilization/activation during tumorigenesis. The COP9 signalosome (CSN) is a protein complex first identified in plant ( Arabidopsis ) mutants that mimic light-induced seedling development when grown in the dark (photomorphogenesis) [1] , [2] , [3] , [4] . CSN is an evolutionarily conserved multiprotein complex involved in protein degradation, and is implicated in signal transduction [5] , [6] , cell cycle [7] , [8] , [9] , transcriptional activation [4] , [10] and tumorigenesis [9] , [11] , [12] , [13] , [14] , [15] , [16] , [17] . Nonetheless, the detailed biological functions of CSN subunits remain unclear. CSN employs its activity towards Cullin-Ring ubiquitin ligases (CRLs) [18] , [19] , thereby coordinating CRL-mediated ubiquitination activity. For example, SCF (Skp1-Cullin-F-box) ubiquitin ligases are CRLs that target many proteins for ubiquitin-mediated degradation [20] . Importantly, Cullin is modified by Nedd8 (ref. 21 ), and this modification (that is, neddylation) is important for the activity of CRLs [22] . A deneddylation process can remove Nedd8 from Cullin [5] . The removal of Nedd8 is catalysed by CSN subunit 5 (CSN5) via linking of its JAMM (JAB1/MPN/Mov34) motif to the metalloprotease activity [6] that can deneddylate Cullin [5] , [22] , [23] , [24] . So far, the molecular mechanism of other subunit’s involvement in regulating CRL activity remains unresolved. The CSN1, 2, 3, 4, 7 and 8 subunits each contain a PCI (Proteasome, COP9 signalosome, translation initiation factor) domain, which may serve as a scaffold in the assembly of the CSN. The CSN6 and CSN5 subunits each contain an MPN domain [6] , [25] , [26] , [27] . The MPN domain of CSN5 is involved in deneddylating Cullin [6] . Although the MPN domain of CSN6 is 70% homologous to that of CSN5, the biochemical function of the CSN6 MPN domain has yet to be defined. In fission yeast genetic studies, neither Csn4- nor Csn5-null mutants have phenotypes similar to those of Csn1- and Csn2-null mutants, suggesting that different subunits of the CSN mediate distinct functions [28] , [29] . We expect that CSN6’s role is unique. Our CSN6 knockout study [15] provided an important research tool for further addressing CSN6’s biological role in terms of CRL regulation. Amplification of the CSN6 gene was detected in a high percentage of breast cancer samples [15] . Analysing human cancer patient transcriptomic data sets further revealed that overexpression of CSN6 in cancer is a common phenomenon [13] . Thus, CSN6 has emerging roles in cancer. However, the mechanistic impact of CSN6 in cancer has not been well characterized. Myc can induce tumorigenesis by promoting cell proliferation and blocking cell differentiation [30] . Modest overexpression of Myc disrupts DNA-damage checkpoint control [31] , [32] , resulting in genomic instability and tumour progression [33] . Myc levels need to be tightly regulated to abrogate Myc’s unfavourable impact. However, the mechanism by which the Myc protein level is regulated is not well characterized. Peptidyl-prolyl isomerase (Pin1) recognizes the phosphorylated Thr 58-Pro motif of Myc and facilitates the subsequent degradation of Myc [34] by ubiquitin ligase Fbxw7 (refs 35 , 36 ). Although Fbxw7 is involved in regulating Myc stability, the upstream regulator of the Fbxw7 has yet to be investigated. We find that CSN6-enhanced Cullin neddylation facilitates autoubiquitination and degradation of Myc E3 ligase Fbxw7, thereby stabilizing Myc which indicates that CSN6 is a positive upstream regulator of Myc. Our studies on the CSN6–Cullin–Fbxw7–Myc axis signal regulation reported here fill important knowledge gaps concerning roles of CSN6 in Cullin neddylation regulation, Fbxw7 ubiquitination and Myc stabilization/activation in human cancer. Loss of CSN6 decreases Myc transcriptional activity We have generated mice carrying a targeted disruption of the Csn6 gene [15] . Although homozygous deletion of Csn6 in mice causes early embryonic lethality, loss of one Csn6 allele does not [15] . To explore the signalling pathways regulated by CSN6, we compared the protein expression profiles of Csn6 +/− and Csn6 +/+ mouse embryonic fibroblasts (MEFs). Csn6 +/− MEFs showed a lower level of CSN6 protein, as expected, but demonstrated no reductions of CSN5, CSN7 or CSN8 levels compared with Csn6 +/+ MEFs ( Fig. 1a ). Importantly, the levels of neddylated Cullin-1 and Cullin-4A were lower in Csn6 +/− MEFs than in Csn6 +/+ MEFs ( Fig. 1a ; Supplementary Fig. 1a ). Investigation of other oncogenes and tumour suppressors related to cell growth showed that c-Myc (hereafter Myc), CDK4, p21, p27 and p53 levels were different in Csn6 +/− MEFs than in Csn6 +/+ MEFs ( Fig. 1a ). 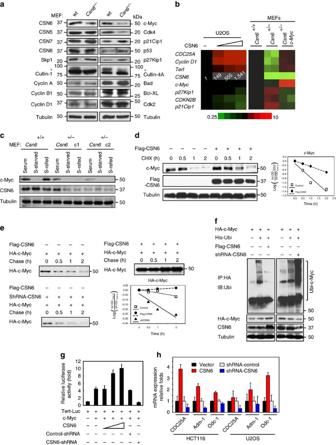Figure 1: Loss of CSN6 leads to destabilization of Myc and decreases Myc transcriptional activity. (a) Immunoblot analysis ofCsn6+/−MEFs. Primary MEF cells were prepared from 13.5-day embryos derived from wild-type (wt)Csn6+/+andCsn6+/−mice. After 4 days of culture, cell lysates were analysed by indicated antibodies. (b) Quantitative RT–PCR analysis of mRNA levels for indicated c-Myc target genes in CSN6-transfected U2OS cells orCsn6+/−MEFs. The quantitated mRNA expression level was normalized toGAPDHmRNA. Two MEFs were examined for each genotype. Expression level of transfected CSN6 is indicated as numbers on the heat map, and the heat map depicts the natural logarithm of fold-change in mRNA expression. (c) CSN6 knockdown abrogated serum-induced elevation of Myc.Csn6+/+MEFs andCsn6+/−clone 1 (C1) and clone 2 (C2) MEFs were serum-starved for 24 h and then were refed with serum for 24 h. Lysates were analysed by indicated antibodies. (d) CSN6 decreased Myc turnover. 293T cells were transfected with Flag-CSN6 and were then treated with cycloheximide (CHX; 100 μg ml−1) for the indicated times. The immunoblot of the Myc signal at each time point was measured using a densitometer and the integrated optical density of Myc was measured. The turnover of Myc is indicated graphically. (e) CSN6 expression affected Myc turnover.35S–pulse-labelled HA-Myc protein was immunoprecipitated from indicated transfected 293T cell lysates. The mixture was separated by SDS polyacrylamide gel electrophoresis (PAGE) and the gel was exposed to an X-ray film. The density of HA-Myc was measured and the integrated optical density (OD) was measured. The turnover of HA-Myc is indicated graphically. (f) CSN6 decreased ubiquitination levels of Myc. 293T cells were transfected with indicated plasmids. Cells were treated with 50 μg ml−1MG132 for 6 h before harvest. The ubiquitinated Myc proteins were pulled down with anti-HA antibody and immunoblotted with anti-ubiquitin (Ubi) antibody. (g) CSN6 activated Myc transcriptional activity. The Tert-luc reporter containing a Myc response element (Ebox) was transfected with the Myc-expressing vectors and increasing amounts of the CSN6 expression vector or CSN6 shRNA plasmid into 293T cells. Relative luciferase activities are shown with error bars representing s.d. Each result shown is representative of three independent experiments. (h) CSN6 elevated expression of Myc target genes. Quantitative real-time RT–PCR analysis of Myc target gene expression, including CDC25A, Adm-1 and ODC-1, in indicated cells. The error bars represent 95% confidence intervals. Each result shown is representative of three independent experiments. Figure 1: Loss of CSN6 leads to destabilization of Myc and decreases Myc transcriptional activity. ( a ) Immunoblot analysis of Csn6 +/− MEFs. Primary MEF cells were prepared from 13.5-day embryos derived from wild-type (wt) Csn6 +/+ and Csn6 +/− mice. After 4 days of culture, cell lysates were analysed by indicated antibodies. ( b ) Quantitative RT–PCR analysis of mRNA levels for indicated c-Myc target genes in CSN6-transfected U2OS cells or Csn6 +/− MEFs. The quantitated mRNA expression level was normalized to GAPDH mRNA. Two MEFs were examined for each genotype. Expression level of transfected CSN6 is indicated as numbers on the heat map, and the heat map depicts the natural logarithm of fold-change in mRNA expression. ( c ) CSN6 knockdown abrogated serum-induced elevation of Myc. Csn6 +/+ MEFs and Csn6 +/− clone 1 (C1) and clone 2 (C2) MEFs were serum-starved for 24 h and then were refed with serum for 24 h. Lysates were analysed by indicated antibodies. ( d ) CSN6 decreased Myc turnover. 293T cells were transfected with Flag-CSN6 and were then treated with cycloheximide (CHX; 100 μg ml −1 ) for the indicated times. The immunoblot of the Myc signal at each time point was measured using a densitometer and the integrated optical density of Myc was measured. The turnover of Myc is indicated graphically. ( e ) CSN6 expression affected Myc turnover. 35 S–pulse-labelled HA-Myc protein was immunoprecipitated from indicated transfected 293T cell lysates. The mixture was separated by SDS polyacrylamide gel electrophoresis (PAGE) and the gel was exposed to an X-ray film. The density of HA-Myc was measured and the integrated optical density (OD) was measured. The turnover of HA-Myc is indicated graphically. ( f ) CSN6 decreased ubiquitination levels of Myc. 293T cells were transfected with indicated plasmids. Cells were treated with 50 μg ml −1 MG132 for 6 h before harvest. The ubiquitinated Myc proteins were pulled down with anti-HA antibody and immunoblotted with anti-ubiquitin (Ubi) antibody. ( g ) CSN6 activated Myc transcriptional activity. The Tert-luc reporter containing a Myc response element (Ebox) was transfected with the Myc-expressing vectors and increasing amounts of the CSN6 expression vector or CSN6 shRNA plasmid into 293T cells. Relative luciferase activities are shown with error bars representing s.d. Each result shown is representative of three independent experiments. ( h ) CSN6 elevated expression of Myc target genes. Quantitative real-time RT–PCR analysis of Myc target gene expression, including CDC25A, Adm-1 and ODC-1, in indicated cells. The error bars represent 95% confidence intervals. Each result shown is representative of three independent experiments. Full size image The reduced level of Myc in Csn6 +/− MEFs suggested that CSN6 might be important for Myc stabilization. Because Myc is expressed ubiquitously during embryogenesis and is required for mouse embryonic development [37] , we focused on Myc and examined whether CSN6 regulates Myc-mediated transcriptional activity. We examined the expression of Myc targets in Csn6 +/− MEFs and CSN6-overexpressing U2OS cells by real-time quantitative reverse transcriptase PCR (qRT–PCR) ( Fig. 1b ). Overexpression of CSN6 increased the messenger RNA (mRNA) levels of Myc transcriptional targets ( CDC25A , cyclin D1 and Tert ) and decreased the mRNA levels of Myc transcriptionally repressed genes ( p27Kip1 , CDKN2B and p21Cip1 ), while loss of CSN6 reversed the expression of these Myc target genes. Rescued Myc by overexpressing Myc in Csn6 +/− MEFs revealed increased mRNA levels of Myc transcriptional targets and decreased mRNA levels of Myc transcriptionally repressed genes. The data indicate that CSN6 expression can alter Myc-mediated gene regulation. CSN6 increases Myc stability by reducing Myc ubiquitination QRT–PCR data indicating that CSN6 status did not affect Myc mRNA levels ( Fig. 1b ) suggested that CSN6 may regulate Myc levels post-transcriptionally. Myc plays a key role during the G0/G1 to S phase transition. Serum starvation and serum refeeding lead cell cycles transit from quiescent G0 phase to traverse G1 phase and enter the S phase with the induction of Myc expression. Myc was elevated in Csn6 +/+ MEFs by serum refeeding after serum starvation ( Fig. 1c ), but Myc elevation was abrogated in Csn6 +/− MEFs ( Fig. 1c ), thereby reducing cell proliferation ( Supplementary Fig. 1b,c ). These data suggested that the stability and activity of endogens Myc in Csn6 +/− might be disrupted due to loss of one copy of the Csn6 gene. Compared with empty vector-transfected control cells, cells transfected with CSN6 had a decelerated endogenous Myc turnover rate ( Fig. 1d ); the pulse-chase analyses of overexpressed Myc with CSN6 or with short hairpin RNA (shRNA)-mediated CSN6 knockdown indicated that overexpression of CSN6 stabilized Myc while shRNA-CSN6 increased Myc degradation ( Fig. 1e ). Because Myc is degraded through the ubiquitin pathway [38] , we examined whether ubiquitination is involved and found that CSN6 overexpression inhibited Myc ubiquitination while shRNA-CSN6 increased Myc ubiquitination ( Fig. 1f ). CSN6-mediated Myc stabilization translated to increased Myc transcriptional activity, as evidenced by increasing Myc luciferase reporter gene activity ( Fig. 1g ) and qRT–PCR for expression of Myc target genes, including CdC25A, Adm-1 and Odc-1 ( Fig. 1h ). While CSN6 expression increased Myc transcriptional activity, CSN6 knockdown by shRNA reduced Myc transcriptional activity ( Fig. 1h ). CSN6 regulates the SCF–Fbxw7 complex to stabilize Myc SCF ubiquitin ligases target many proteins for ubiquitin-mediated degradation [20] . Modification of Cullins with Nedd8 (neddylation) is important for the activity of CRLs [22] . To further investigate how CSN6 regulates Myc ubiquitination, we examined the major Myc E3 ligase Fbxw7 (refs 11 , 39 , 40 ) and its complex adaptor Cullin-1. First, we found that CSN6 associated with Myc, Fbxw7 and Cullin-1 in U2OS cells in vivo ( Fig. 2a ), suggesting that CSN6 interacts with the SCF complex and may regulate it to stabilize Myc. Knockdown of CSN6 by shRNA led to reduction of Cullin-1 neddylation ( Fig. 2b ). This reduction of Cullin-1 neddylation was accompanied by increased association between Cullin-1 and CAND1, which binds to Cullin-1 when Cullin-1 is not neddylated ( Fig. 2b ). We then found that increasing amounts of CSN6 enhanced neddylation of wild-type (wt) Cullin-1, but not the Cullin-1 mutant [41] , in which the Nedd-8–conjugating site lysine (K) 720 was mutated to arginine (R) ( Supplementary Fig. 2a ). Cullin-1 neddylation was rescued in Csn6 +/− MEFs by treatment of o-phenathroline, a zinc chelator and inhibitor of deneddylation ( Supplementary Fig. 2b ). These data demonstrate that CSN6 is a positive factor for Cullin-1 neddylation. 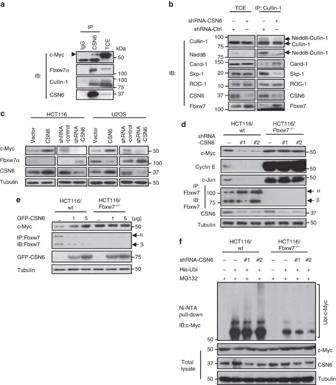Figure 2: CSN6 regulates the SCF (Skp1/Cullin-1/Fbxw7) complex to stabilize Myc. (a) CSN6 associated with Myc, Fbxw7 and Cullin-1. The U2OS cell lysates were immunoprecipitated with anti-CSN6 and immunoblotted with indicated antibodies. (b) CSN6 knockdown led to decreased Cullin-1 neddylation. The U2OS cell lysates were immunoprecipitated with anti-Cullin-1, followed by immunoblotting with indicated antibodies. (c) CSN6 expression was inversely related to Fbxw7 expression. Immunoblot analysis of Myc and Fbxw7α in CSN6-overexpressing or CSN6 knockdown cells. Cell lysates were analysed by indicated antibodies. (d) Knockdown of CSN6 increased the expression of Fbxw7 and reduced Myc. Indicated cells were infected with lentivirus to express one of two independent CSN6 shRNAs (#1 and #2) or luciferase control shRNA. Cell lysates were immunoblotted with indicated antibodies. (e) CSN6 reduced steady-state expression of Fbxw7 to upregulate Myc. Indicated cells were transfected with increasing amounts of GFP-CSN6. Cell lysates were immunoblotted with indicated antibodies. Fbxw7α and Fbxw7β isoforms were identified. (f) Knockdown of CSN6 enhanced Myc ubiquitination. Indicated cells were infected with lentivirus to express one of two independent CSN6 shRNAs (#1 and #2) or luciferase control shRNA. The cells were then transfected with His-ubiquitin and treated with MG132 for 6 h before harvest. The ubiquitinated Myc proteins were pulled down using Ni-NTA-agarose beads and detected with anti-Myc antibody. Figure 2: CSN6 regulates the SCF (Skp1/Cullin-1/Fbxw7) complex to stabilize Myc. ( a ) CSN6 associated with Myc, Fbxw7 and Cullin-1. The U2OS cell lysates were immunoprecipitated with anti-CSN6 and immunoblotted with indicated antibodies. ( b ) CSN6 knockdown led to decreased Cullin-1 neddylation. The U2OS cell lysates were immunoprecipitated with anti-Cullin-1, followed by immunoblotting with indicated antibodies. ( c ) CSN6 expression was inversely related to Fbxw7 expression. Immunoblot analysis of Myc and Fbxw7α in CSN6-overexpressing or CSN6 knockdown cells. Cell lysates were analysed by indicated antibodies. ( d ) Knockdown of CSN6 increased the expression of Fbxw7 and reduced Myc. Indicated cells were infected with lentivirus to express one of two independent CSN6 shRNAs (#1 and #2) or luciferase control shRNA. Cell lysates were immunoblotted with indicated antibodies. ( e ) CSN6 reduced steady-state expression of Fbxw7 to upregulate Myc. Indicated cells were transfected with increasing amounts of GFP-CSN6. Cell lysates were immunoblotted with indicated antibodies. Fbxw7α and Fbxw7β isoforms were identified. ( f ) Knockdown of CSN6 enhanced Myc ubiquitination. Indicated cells were infected with lentivirus to express one of two independent CSN6 shRNAs (#1 and #2) or luciferase control shRNA. The cells were then transfected with His-ubiquitin and treated with MG132 for 6 h before harvest. The ubiquitinated Myc proteins were pulled down using Ni-NTA-agarose beads and detected with anti-Myc antibody. Full size image The Skp1/Cullin-1/F-box complex has two types of ubiquitin ligases, Fbxw7 and Skp2 (refs 32 , 33 ), which are involved in Myc degradation. Interestingly, CSN6 decreased expression of both Fbxw7α and Skp2 ( Supplementary Fig. 3a–c ) with concurrent elevation of Myc. Overexpression of CSN6 reduced the protein levels of Fbxw7α and increased Myc protein levels; while CSN6 knockdown by shRNA resulted in increased protein levels of Fbxw7α and decreased protein levels of Myc in two cell lines HCT116 and U2OS cells ( Fig. 2c ). Knockdown of CSN6 decreased the steady-state expression of Myc protein in HCT116 Fbxw7 +/+ , but not in HCT116 Fbxw7 −/− cells ( Fig. 2d ). Accordingly, CSN6-mediated Myc increases occurred only in HCT116 Fbxw7 +/+ cells ( Fig. 2e ). However, CSN6 shRNA-mediated Myc destabilization still occurred in Skp2-null MEFs ( Supplementary Fig. 3d ), indicating that Skp2 is not critical for the regulation of Myc by CSN6. Furthermore, Fbxw7 deficiency compromised CSN6 shRNA-enhanced Myc ubiquitination ( Fig. 2f ), suggesting that CSN6-mediated Myc stabilization is dependent on Fbxw7. CSN6 enhances Fbxw7’s autoubiquitination and degradation Given these results that Fbxw7 is critical for the regulation of Myc by CSN6, we then focused on Fbxw7. Consistently, CSN6 knockdown decreased turnover rate of Fbxw7 ( Fig. 3a ; Supplementary Fig. 4a ). CSN6-mediated downregulation of Fbxw7 was inhibited by MG132, a 26S proteasome inhibitor ( Fig. 3b ). Notably, Fbxw7 mRNA level was not affected by increasing amounts of CSN6 in several cell lines ( Supplementary Fig. 4b ), suggesting that CSN6 regulates Fbxw7 levels post-transcriptionally. We found that ectopic expression of CSN6 increased the amount of polyubiquitinated Fbxw7α ( Fig. 3c ). Importantly, CSN6 used wt ubiquitin His-Ubi or His-Ubi K63R mutant to cause further ubiquitination of Fbxw7 but was unable to employ His-Ubi K48R mutant to enhance Fbxw7 ubiquitination ( Fig. 3c ), indicating that CSN6-mediated ubiquitination of Fbxw7 is a K48 linkage ( Fig. 3c ), which generally targets proteins for degradation [42] . 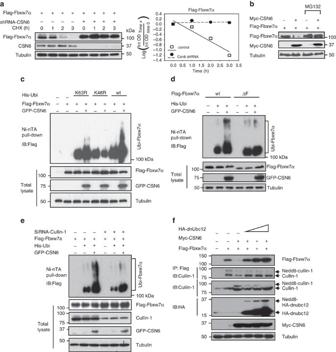Figure 3: CSN6 enhances Fbxw7’s autoubiquitination and degradation. (a) CSN6 increased Fbxw7α turnover. 293T cells were infected with lentivirus to express CSN6 shRNA or luciferase control shRNA. The cells were then transfected with Flag-Fbxw7α and were then treated with cycloheximide (CHX; 100 μg ml−1) for the indicated times. The density of Fbxw7α was measured and the integrated optical density (OD) was measured. The turnover of Fbxw7α is indicated graphically. (b) CSN6-mediated Fbxw7α downregulation was proteasome dependent. 293T cells were cotransfected with indicated plasmids and were treated with or without 50 μg ml−1MG132 for 6 h. The cell lysates were then immunoblotted with the indicated antibodies. (c) CSN6 enhanced Fbxw7α ubiquitination through lysine 48 linkage. 293T cells were cotransfected with Flag-Fbxw7α with or without GFP-CSN6 plus His-ubiquitin wild type (wt), K63R mutant or K48R mutant. Cells were treated with 50 μg ml−1MG132 for 6 h before harvest. The ubiquitinated Fbxw7α proteins were pulled down using Ni-NTA-agarose beads and detected with anti-Flag antibody. (d) An F-box domain deletion mutant of Fbxw7α was resistant to CSN6-mediated ubiquitination. 293T cells were cotransfected with GFP-CSN6, His-ubiquitin plus Flag-Fbxw7α wild-type or F-box domain deletion mutant (ΔF). Cells were treated with 50 μg ml−1MG132 for 6 h before harvest. The ubiquitinated Fbxw7α proteins were pulled down using Ni-NTA-agarose beads and detected with anti-Flag antibody. (e) Cullin-1 knockdown diminished CSN6-induced ubiquitination of Fbxw7α. 293T cells were transfected with siRNA Cullin-1 or siRNA control plus indicated plasmids. Cells were treated with 50 μg ml−1MG132 for 6 h before harvest. The ubiquitinated Fbxw7α proteins were pulled down using Ni-NTA-agarose beads and detected with anti-Flag antibody. (f) Cullin-1 neddylation was involved in CSN6-mediated downregulation of Fbxw7α. 293T cells were transfected with indicated plasmids plus increasing amounts of HA-dnUbc12. The levels of Nedd8-Cullin-1 and Nedd8-dnUbc12 were detected with anti-Nedd8 antibody. Figure 3: CSN6 enhances Fbxw7’s autoubiquitination and degradation. ( a ) CSN6 increased Fbxw7α turnover. 293T cells were infected with lentivirus to express CSN6 shRNA or luciferase control shRNA. The cells were then transfected with Flag-Fbxw7α and were then treated with cycloheximide (CHX; 100 μg ml −1 ) for the indicated times. The density of Fbxw7α was measured and the integrated optical density (OD) was measured. The turnover of Fbxw7α is indicated graphically. ( b ) CSN6-mediated Fbxw7α downregulation was proteasome dependent. 293T cells were cotransfected with indicated plasmids and were treated with or without 50 μg ml −1 MG132 for 6 h. The cell lysates were then immunoblotted with the indicated antibodies. ( c ) CSN6 enhanced Fbxw7α ubiquitination through lysine 48 linkage. 293T cells were cotransfected with Flag-Fbxw7α with or without GFP-CSN6 plus His-ubiquitin wild type (wt), K63R mutant or K48R mutant. Cells were treated with 50 μg ml −1 MG132 for 6 h before harvest. The ubiquitinated Fbxw7α proteins were pulled down using Ni-NTA-agarose beads and detected with anti-Flag antibody. ( d ) An F-box domain deletion mutant of Fbxw7α was resistant to CSN6-mediated ubiquitination. 293T cells were cotransfected with GFP-CSN6, His-ubiquitin plus Flag-Fbxw7α wild-type or F-box domain deletion mutant (ΔF). Cells were treated with 50 μg ml −1 MG132 for 6 h before harvest. The ubiquitinated Fbxw7α proteins were pulled down using Ni-NTA-agarose beads and detected with anti-Flag antibody. ( e ) Cullin-1 knockdown diminished CSN6-induced ubiquitination of Fbxw7α. 293T cells were transfected with siRNA Cullin-1 or siRNA control plus indicated plasmids. Cells were treated with 50 μg ml −1 MG132 for 6 h before harvest. The ubiquitinated Fbxw7α proteins were pulled down using Ni-NTA-agarose beads and detected with anti-Flag antibody. ( f ) Cullin-1 neddylation was involved in CSN6-mediated downregulation of Fbxw7α. 293T cells were transfected with indicated plasmids plus increasing amounts of HA-dnUbc12. The levels of Nedd8-Cullin-1 and Nedd8-dnUbc12 were detected with anti-Nedd8 antibody. Full size image Fbxw7 is rapidly ubiquitinated and degraded by an autocatalytic mechanism that is dependent upon its ability to interact with the SCF components Cullin-1 and Skp1 (ref. 43 ). We showed that the F-box deletion mutant of Fbxw7α, which has reduced binding to Cullin-1 and Skp1 ( Supplementary Fig. 5a–c ), was more resistant to CSN6-induced degradation ( Supplementary Fig. 5d ) and ubiquitination ( Fig. 3d ) than wt Fbxw7α. It is important to point out that CSN6 interacted with all the three isoforms of Fbxw7 (refs 44 , 45 ) and reduced the steady-state expression of Fbxw7 in a dose-dependent manner ( Supplementary Fig. 6a–c ). In vitro ubiquitination assays also showed that CSN6 enhanced Fbxw7 ubiquitination and diminished Fbxw7-mediated ubiquitinations of Fbxw7’s targets, Myc and cyclin E ( Supplementary Fig. 6d–f ). Neddylation of Cullin-1 can affect CRL substrate adaptors through autocatalytic degradation [18] . We next addressed whether Cullin-1 is involved in CSN6-mediated Fbxw7 downregulation. We found that knockdown of Cullin-1 compromised CSN6-induced ubiquitination of Fbxw7 ( Fig. 3e ). We further showed that overexpression of dominant-negative Ubc12 (dn-Ubc12-HA) [46] , [47] , which antagonized CSN6-mediated increase of Cullin-1 neddylation, compromised CSN6-mediated Fbxw7α downregulation ( Fig. 3f ). These data demonstrate that Cullin-1 and its neddylation are critical for CSN6-mediated Fbxw7 downregulation and ubiquitination. Together, these data suggest that CSN6-mediated Fbxw7 autoubiquitination involved the SCF complex. CSN6 competes with CSN5 to increase Cullin neddylation We examined gel-filtration chromatography fractions from spleen extracts from Csn6 +/+ and Csn6 +/− mice and found that Csn6 +/− cell extracts had more non-neddylated forms of Cullin-1 than Csn6 +/+ cell extracts when compared side by side ( Fig. 4a,b ), suggesting that CSN6 is preserving Cullin-1 neddylation. We found that both CSN6 and CSN5 associated with Cullin-1 and that CSN6 and CSN5 competed with each other for Cullin-1 binding in a dose-dependent manner ( Fig. 4c ). Consequently, increasing CSN6 expression increased its competition with CSN5, preventing CSN5-mediated deneddylation of Cullin-1 and thereby increasing neddylation of Cullin-1 in a dose-dependent manner ( Fig. 4c ). Increasing CSN5, on the other hand, increased competition with CSN6 for Cullin-1 binding, thereby decreasing Cullin-1 neddylation ( Fig. 4c ). The gel-filtration analyses performed in overexpressed CSN6 HCT116 cells also support this important role of the ratios of CSN5/CSN6 in the CSN complex in determining Cullin neddylation levels ( Supplementary Fig. 7 ). 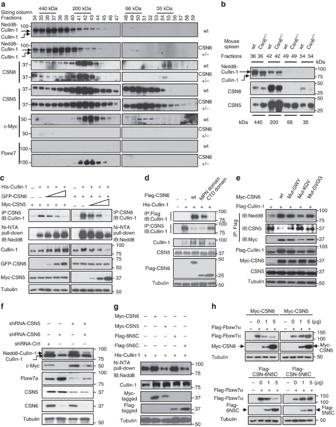Figure 4: CSN6 enhances neddylation of Cullin-1 via its MPN domain. (a) Neddylation status of Cullin in gel-filtration chromatography fractions from spleen extracts fromCsn6+/+(wt) andCsn6+/−mice. Extracts of spleen from CSN6+/+orCsn6+/−mice (4 weeks old) were ground and subjected to lysis. Lysates were fractionated by gel-filtration chromatography. Fractions were resolved by SDS-PAGE, followed by immunoblotting with indicated antibodies. Molecular size of eluted fraction is indicated above. (b) Non-neddylated Cullin was increased inCsn6+/−mice. Extracts of spleen from CSN6+/+(wt) orCsn6+/−mice were fractionated by gel filtration chromatography. Representative fractions 36–54 from (a) were resolved by SDS-polyacrylamide gel electrophoresis, followed by immunoblotting with anti-Cullin-1, anti-CSN6 and anti-CSN5 antibodies. (c) CSN6 competed with CSN5 for binding to Cullin-1 and affected Cullin-1 neddylation. 293T cells were transfected with His-Cullin-1 plus increasing amounts of GFP-CSN6 or Myc-CSN5. The neddylated Cullin-1 proteins were pulled down using Ni-NTA-agarose beads and detected with anti-Nedd8 antibody. The lysates were also immunoprecipitated with CSN6 antibody or CSN5 antibody and were subjected to immunoblotting with anti-Cullin-1. (d) MPN domain of CSN6 had an important role in competing with CSN5 for Cullin-1 binding and affected Cullin-1 neddylation. 293T cells were cotransfected with indicated plasmids. The lysates were immunoprecipitated with anti-Flag or anti-CSN5 antibody and immunoblotted with the indicated antibodies. (e) Mutation of conserved residues in the MPN domain of CSN6 compromised CSN6’s capacity for competing with CSN5. 293T cells were cotransfected with indicated CSN6 MPN mutant plasmids. The lysates were immunoprecipitated with anti-Flag antibody and immunoblotted with indicated antibodies. (f) CSN6 antagonized CSN5 in regulating Cullin-1 neddylation. U2OS cells were infected with the indicated lentivirus carrying CSN6 shRNA, CSN5 shRNA or luciferase control shRNA. Cell lysates were immunoblotted with the indicated antibodies. (g) The chimeric protein 6N5C expressing the CSN6 MPN domain functioned like wild-type CSN6 in increasing Cullin-1 neddylation. 293T cells were cotransfected with indicated wild-type- and chimeric protein-expressing plasmids. The lysates were pulled down with Ni-NTA-agarose beads and immunoblotted with anti-Nedd8. (h) Both chimeric protein 6N5C and wild-type CSN6 decreased the stability of Fbxw7α in a dose-dependent manner. 293T cells were cotransfected with indicated plasmids. The lysates were immunoblotted with indicated antibodies. Figure 4: CSN6 enhances neddylation of Cullin-1 via its MPN domain. ( a ) Neddylation status of Cullin in gel-filtration chromatography fractions from spleen extracts from Csn6 +/+ (wt) and Csn6 +/− mice. Extracts of spleen from CSN6 +/+ or Csn6 +/− mice (4 weeks old) were ground and subjected to lysis. Lysates were fractionated by gel-filtration chromatography. Fractions were resolved by SDS-PAGE, followed by immunoblotting with indicated antibodies. Molecular size of eluted fraction is indicated above. ( b ) Non-neddylated Cullin was increased in Csn6 +/− mice. Extracts of spleen from CSN6 +/+ (wt) or Csn6 +/− mice were fractionated by gel filtration chromatography. Representative fractions 36–54 from ( a ) were resolved by SDS-polyacrylamide gel electrophoresis, followed by immunoblotting with anti-Cullin-1, anti-CSN6 and anti-CSN5 antibodies. ( c ) CSN6 competed with CSN5 for binding to Cullin-1 and affected Cullin-1 neddylation. 293T cells were transfected with His-Cullin-1 plus increasing amounts of GFP-CSN6 or Myc-CSN5. The neddylated Cullin-1 proteins were pulled down using Ni-NTA-agarose beads and detected with anti-Nedd8 antibody. The lysates were also immunoprecipitated with CSN6 antibody or CSN5 antibody and were subjected to immunoblotting with anti-Cullin-1. ( d ) MPN domain of CSN6 had an important role in competing with CSN5 for Cullin-1 binding and affected Cullin-1 neddylation. 293T cells were cotransfected with indicated plasmids. The lysates were immunoprecipitated with anti-Flag or anti-CSN5 antibody and immunoblotted with the indicated antibodies. ( e ) Mutation of conserved residues in the MPN domain of CSN6 compromised CSN6’s capacity for competing with CSN5. 293T cells were cotransfected with indicated CSN6 MPN mutant plasmids. The lysates were immunoprecipitated with anti-Flag antibody and immunoblotted with indicated antibodies. ( f ) CSN6 antagonized CSN5 in regulating Cullin-1 neddylation. U2OS cells were infected with the indicated lentivirus carrying CSN6 shRNA, CSN5 shRNA or luciferase control shRNA. Cell lysates were immunoblotted with the indicated antibodies. ( g ) The chimeric protein 6N5C expressing the CSN6 MPN domain functioned like wild-type CSN6 in increasing Cullin-1 neddylation. 293T cells were cotransfected with indicated wild-type- and chimeric protein-expressing plasmids. The lysates were pulled down with Ni-NTA-agarose beads and immunoblotted with anti-Nedd8. ( h ) Both chimeric protein 6N5C and wild-type CSN6 decreased the stability of Fbxw7α in a dose-dependent manner. 293T cells were cotransfected with indicated plasmids. The lysates were immunoblotted with indicated antibodies. Full size image Our data revealed that the MPN domain of CSN6, but not the C-terminal domain of CSN6, interacted with Cullin-1 ( Fig. 4d ). Notably, the MPN domain of CSN6 inhibited the association of CSN5 with Cullin-1, while the C-terminal domain had less impact ( Fig. 4d ). To further understand the mechanism behind this Cullin-1-binding competition, we constructed several MPN mutants of CSN6 by mutating residues conserved between CSN5 and CSN6, including MPN-GVGG (63G, 68V, 70G, 74G→AAAA), MPN-KQV (113K, 114Q, 115V→AAA) and MPN-GWY (123G, 124W, 125Y→AAA) ( Fig. 4e ; Supplementary Fig. 8a,b ). We found these CSN6 mutants compromised their competitive activity in preventing binding between CSN5 and Cullin-1 when compared with wt CSN6; therefore, their capacity to interfere with endogenous CSN5-mediated deneddylation of Cullin-1 was also altered ( Fig. 4e ). Thus, some conserved MPN residues of CSN6 are critical for its competition with CSN5 in terms of Cullin-1 association. CSN6 MPN facilitates Cullin neddylation to regulate Fbxw7 We then knocked down CSN6 or CSN5 to examine the correlation between Cullin-1 neddylation and regulation of Myc and Fbxw7 stability ( Fig. 4f ). CSN6 knockdown reduced the neddylated form of Cullin-1, leading to accumulation of Fbxw7, which in turn caused downregulation of Myc ( Fig. 4f ). In contrast, CSN5 knockdown led to accumulation of the neddylated form of Cullin-1 and destabilization of Fbxw7, causing accumulation of Myc ( Fig. 4f ). Compared with wt CSN6, which clearly decreased Fbxw7 expression and increased Myc expression in U2OS cells, the MPN-KQV CSN6 mutant lost these functions ( Supplementary Fig. 8c–e ). To further characterize the contribution of the MPN domain of CSN6 in regulating Cullin neddylation, we constructed two chimeric proteins: one comprising CSN6’s N-terminal domain containing the MPN motif fused with CSN5’s C-terminal domain (called myc-tagged 6N5C), the other comprising CSN5’s N-terminal domain containing the MPN motif fused with CSN6’s C-terminal domain (called myc-tagged 5N6C). We then performed the Cullin neddylation assay with each protein ( Fig. 4g ). Both wt CSN6 and myc-tagged 6N5C increased Cullin-1 neddylation, while both wt CSN5 and myc-tagged 5N6C reduced Cullin-1 neddylation ( Fig. 4g ), suggesting that the MPN domain of CSN6 functions differently from that of CSN5 and is the critical region for facilitation of Cullin-1 neddylation. This CSN6–Cullin relationship translated into decreasing steady-state expression of Fbxw7, as evidenced by the observation that both wt CSN6 and Myc-tagged 6N5C decreased the stability of Fbxw7, while both wt CSN5 and Myc-tagged 5N6C increased the steady-state expression of Fbxw7 ( Fig. 4h ). Together, these data suggest that CSN6 increases Cullin-1 neddylation by competing with CSN5 for binding to Cullin-1 through the MPN domain, thereby facilitating Cullin-1-enhanced Fbxw7 degradation. CSN6 deficiency compromises Myc target gene expression The oncogenic role of Myc is documented in the Eμ- Myc transgenic mouse, which develops preB/B-cell lymphomas [48] , [49] . We have shown that CSN6 increases Myc stability. To address the biological significance behind this regulation in vivo , we crossed Csn6 +/− mice to Eμ- Myc transgenic mice. Four-week-old Eμ- Myc/Csn6 +/− mice showed marked reduction of splenomegaly, one of the earliest manifestations of Myc-induced lymphomagenesis, when compared with Eμ- Myc/Csn6 +/+ mice littermates ( Fig. 5a ). These data suggest that Csn6 heterozygosity may delay the onset of Myc-induced B-cell lymphomas. To further examine this idea, B-cell proliferation and apoptosis in the Eμ-Myc mice were monitored by bromodeoxyuridine (BrdU) incorporation and annexin V staining. Eμ- Myc/Csn6 +/− mice had significantly less BrdU incorporation ( Fig. 5b ) and apoptosis than Eμ- Myc/Csn6 +/+ mice ( Fig. 5c ), suggesting that Csn6 heterozygosity impairs Myc-mediated proliferation and apoptosis of pre-tumoral B cells in Eμ- Myc mice. 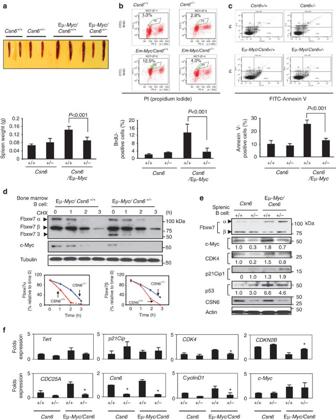Figure 5: Loss of CSN6 compromises lymphomagenesis in the Eμ-Myctransgenic mouse by increasing Fbxw7 stability. (a)Csn6haplo-insufficiency delayed splenomegaly in 4-week-old Eμ-Myc/Csn6+/−mice. Average spleen weights of each group are shown in the bar graph (n=6 per genotype). Representative photographs of littermate mice are shown. Error bars represent 95% confidence intervals (CIs). (b)Csn6haplo-insufficiency reduced the proliferation rate of B cells. 5-bromodeoxyuridine (BrdU) incorporation was measured in splenic B220+ cells (n=3 per genotype). B cells were isolated from the spleens of each group of mice 12 h after injection of BrdU (0.04 μg kg−1). B220+ cells were isolated and stained with fluorescein isothiocyanate (FITC)-conjugated anti-BrdU-antibody, followed by flow cytometric analysis. Representative images of each group of mice are shown. Percentages of BrdU-positive cells are presented (mean±95% CI). (c)Csn6haplo-insufficiency impaired Myc-induced apoptosis in spleen-derived B cells. Flow cytometric analysis was used to measure Myc-induced apoptosis in splenic B220+ cells (n=3 per genotype). B220+ cells were isolated and stained with annexin V. Representative images of each group of mice are shown. Percentages of annexin V-positive cells are presented (mean±95% CI). (d)Csn6haplo-insufficiency reduced turnover of Fbxw7 in B cells from bone marrow. Primary bone marrow-derived B cells were isolated and cultured with recombinant murine IL-7 (50 ng ml−1). Percentages of Fbxw7α and Fbxw7β remaining are indicated graphically. (e)Csn6haplo-insufficiency increased Fbxw7 stability and reduced the protein level of Myc, as well as the expression of Myc target genes in B cells. B cells (B220+) isolated from spleens of indicated mice were immunoblotted with the indicated antibodies. (f)Csn6haplo-insufficiency reduced the transcriptional activity of Myc in B cells. B cells (B220+) isolated from spleens of indicated mice (n=3 per genotype) and total RNA was extracted. The mRNA expression of indicated Myc target genes was analysed by qRT–PCR. Error bars represent 95% CI; Studentt-test, *P<0.001. Figure 5: Loss of CSN6 compromises lymphomagenesis in the Eμ- Myc transgenic mouse by increasing Fbxw7 stability. ( a ) Csn6 haplo-insufficiency delayed splenomegaly in 4-week-old Eμ- Myc/Csn6 +/− mice. Average spleen weights of each group are shown in the bar graph ( n =6 per genotype). Representative photographs of littermate mice are shown. Error bars represent 95% confidence intervals (CIs). ( b ) Csn6 haplo-insufficiency reduced the proliferation rate of B cells. 5-bromodeoxyuridine (BrdU) incorporation was measured in splenic B220+ cells ( n =3 per genotype). B cells were isolated from the spleens of each group of mice 12 h after injection of BrdU (0.04 μg kg −1 ). B220+ cells were isolated and stained with fluorescein isothiocyanate (FITC)-conjugated anti-BrdU-antibody, followed by flow cytometric analysis. Representative images of each group of mice are shown. Percentages of BrdU-positive cells are presented (mean±95% CI). ( c ) Csn6 haplo-insufficiency impaired Myc-induced apoptosis in spleen-derived B cells. Flow cytometric analysis was used to measure Myc-induced apoptosis in splenic B220+ cells ( n =3 per genotype). B220+ cells were isolated and stained with annexin V. Representative images of each group of mice are shown. Percentages of annexin V-positive cells are presented (mean±95% CI). ( d ) Csn6 haplo-insufficiency reduced turnover of Fbxw7 in B cells from bone marrow. Primary bone marrow-derived B cells were isolated and cultured with recombinant murine IL-7 (50 ng ml −1 ). Percentages of Fbxw7α and Fbxw7β remaining are indicated graphically. ( e ) Csn6 haplo-insufficiency increased Fbxw7 stability and reduced the protein level of Myc, as well as the expression of Myc target genes in B cells. B cells (B220+) isolated from spleens of indicated mice were immunoblotted with the indicated antibodies. ( f ) Csn6 haplo-insufficiency reduced the transcriptional activity of Myc in B cells. B cells (B220+) isolated from spleens of indicated mice ( n =3 per genotype) and total RNA was extracted. The mRNA expression of indicated Myc target genes was analysed by qRT–PCR. Error bars represent 95% CI; Student t -test, * P <0.001. Full size image Further studies showed that the turnover rate of Fbxw7 isoforms in B cells from bone marrow of Eμ- Myc / Csn 6 +/− mice was lower than that in B cells of Eμ- Myc / Csn 6 +/+ ( Fig. 5d ). Accordingly, Myc protein turnover was faster in Eμ- Myc / Csn 6 +/− mice than in Eμ- Myc / Csn 6 +/+ mice ( Fig. 5d ). We also assessed the expression of Myc and its target genes in splenic B cells of Eμ- Myc/Csn6 +/− mice and found that these cells had a higher level of Fbxw7, which in turn led to downregulation of Myc, than B cells of Eμ- Myc / Csn 6 +/+ mice ( Fig. 5e ). We also examined expression of Myc target genes, including Tert, CDK4, CDC25A, cyclin D1, CDKN2B and p21Cip1, by qRT–PCR and found that expression of many Myc target genes was reduced or compromised in Eμ- Myc/Csn6 +/− mice compared with Eμ- Myc / Csn6 +/+ mice ( Fig. 5f ). These pre-malignant B-cell studies confirmed CSN6’s stimulatory impact on Myc protein level and transcription activity in vivo . Loss of CSN6 hinders lymphomagenesis in the Eμ-Myc mouse We found that Eμ- Myc / Csn6 +/− mice survived longer than Eμ- Myc / Csn6 +/+ littermates ( Fig. 6a ), suggesting that Myc-induced lymphomagenesis is decelerated by Csn6 heterozygosity. To further understand the molecular basis of lymphomagenesis in these Eμ- Myc mice, we analysed the lymphoma tissues obtained from animals at the end of these experiments. Eμ- Myc/Csn6 +/− lymphomas expressed the CSN6 protein at a lower level, which correlated with lower levels of neddylated Cullin-1, than Eμ- Myc/Csn6 +/+ lymphomas ( Fig. 6b ), attesting to the role of CSN6 in maintaining levels of Cullin-1 neddylation. As already described, Cullin-1 neddylation has an impact on the stability of F-box proteins. Therefore, we also analysed the expression levels of Fbxw7 by immunohistochemistry (IHC) in these lymphomas ( Fig. 6c ). Fbxw7 was expressed in a high percentage of Eμ- Myc/Csn6 +/− lymphomas, but was scarcely expressed in Eμ- Myc/Csn6 +/+ lymphomas ( Fig. 6c,d ). Significantly, Myc protein expression in Eμ- Myc / Csn 6 +/− lymphomas was lower than that in Eμ- Myc / Csn6 +/+ lymphomas ( Fig. 6b,d ). As expected, Myc-mediated transcriptional activation target CDK4 and Myc-mediated transcriptional repression targets p27Kip1 and p21Cip1 were deregulated in Eμ- Myc/Csn6 +/− lymphomas compared with Eμ- Myc/Csn6 +/+ lymphomas ( Fig. 6b,d ). IκBα was upregulated in Eμ- Myc/Csn6 +/− lymphomas ( Fig. 6b ), and loss of p53 expression was less frequent in Eμ- Myc/Csn6 +/− lymphomas than in Eμ- Myc/Csn6 +/+ lymphomas ( Fig. 6b,d ). We quantitated the expression of these proteins in tumour tissues (the levels of Fbxw7 were quantitated from its IHC staining) and present the relative fold of protein expression as bar graphs ( Fig. 6d ). Together, these data indicate that the CSN6–Cullin–Fbxw7 axis plays a pivotal role in Myc-induced lymphomagenesis. On the basis of our findings, we developed a model of Myc regulation by CSN6 ( Fig. 6e ). 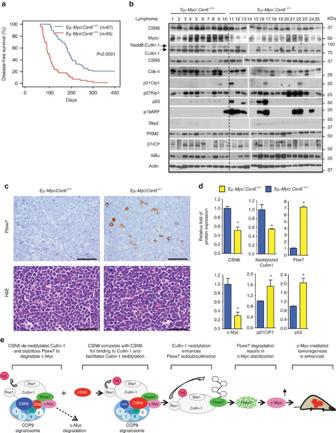Figure 6: CSN6 haplo-insufficiency delays the onset/progression of Myc-mediated lymphomagenesis. (a) Survival of Eμ-Mycmice was prolonged by CSN6 haplo-insufficiency. The genotypes of the transgenic mice are indicated next to the Kaplan–Meier survival curves. The numbers of mice analysed in each group are denoted. (b) CSN6 haplo-insufficiency caused low levels of Cullin neddylation and low expression of Myc. Lymphoma tissues from Eμ-Myc/Csn6+/+(1–10) and Eμ-Myc/Csn6+/−(11–25) mice were immunoblotted with the indicated antibodies. (c) Levels of Fbxw7 were elevated in lymphomas from Eμ-Myc/Csn6+/−mice. Lymphomas arising from mice frombunderwent IHC staining. Representative photographs of Fbxw7 and haematoxylin and eosin staining are shown. Scale bar: 50μm. (d) Levels of neddylated Cullin and Myc were reduced and level of Fbxw7 was increased in lymphomas from transgenic mice. Levels of indicated proteins in lymphomas arising from mice inbandcwere quantitated by integrating optical density from Image J and are demonstrated as bar graphs. Each result shown is representative of three independent experiments. Error bars represent 95% CI; Student’st-test, *P<0.001. (e) The model depicts the pivotal role of the CSN6–Cullin–Fbxw7 axis in Myc-induced lymphomagenesis. Figure 6: CSN6 haplo-insufficiency delays the onset/progression of Myc-mediated lymphomagenesis. ( a ) Survival of Eμ- Myc mice was prolonged by CSN6 haplo-insufficiency. The genotypes of the transgenic mice are indicated next to the Kaplan–Meier survival curves. The numbers of mice analysed in each group are denoted. ( b ) CSN6 haplo-insufficiency caused low levels of Cullin neddylation and low expression of Myc. Lymphoma tissues from Eμ- Myc / Csn6 +/+ (1–10) and Eμ- Myc / Csn6 +/− (11–25) mice were immunoblotted with the indicated antibodies. ( c ) Levels of Fbxw7 were elevated in lymphomas from Eμ- Myc / Csn6 +/− mice. Lymphomas arising from mice from b underwent IHC staining. Representative photographs of Fbxw7 and haematoxylin and eosin staining are shown. Scale bar: 50μm. ( d ) Levels of neddylated Cullin and Myc were reduced and level of Fbxw7 was increased in lymphomas from transgenic mice. Levels of indicated proteins in lymphomas arising from mice in b and c were quantitated by integrating optical density from Image J and are demonstrated as bar graphs. Each result shown is representative of three independent experiments. Error bars represent 95% CI; Student’s t -test, * P <0.001. ( e ) The model depicts the pivotal role of the CSN6–Cullin–Fbxw7 axis in Myc-induced lymphomagenesis. Full size image Deregulation of the CSN6-Myc signalling axis in human cancer CSN6 is amplified/overexpressed in a high percentage of human breast cancer [15] . To understand more about CSN6 overexpression in other types of tumours, we performed transcriptomic analysis of human cancer patient data sets from Oncomine [50] , [51] , [52] as well as Gene Expression Omnibus using Nexus Expression 2.0 and gene set enrichment analysis. We found that CSN6 was overexpressed in >25% of cases of all 11 types of human malignancies examined and in >50% of cases of glioblastoma, pancreatic cancer and breast cancer ( Fig. 7a ). We also showed, using IHC analysis, that this positive relationship between CSN6 and Myc occurred in 123 specimens of human pancreatic cancer collected at the MD Anderson Cancer Center; χ 2 -analysis showed that high Myc expression was significantly ( P <0.001) correlated with high CSN6 expression in these cancer cases ( Supplementary Table 1 ). In tumours in which CSN6 expression was high, Myc expression was high (representative case I in Fig. 7b ), whereas in tumours in which CSN6 expression was low, the Myc signal was low (representative case II in Fig. 7b ). 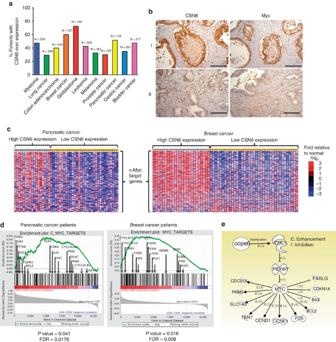Figure 7: CSN6 is overexpressed in many cancer types and correlated with upregulation of Myc target genes. (a) Transcriptomic analysis revealed frequent CSN6 overexpression in human patients with cancer. Human cancer patient data sets were obtained from the Oncomine database and Gene Expression Omnibus. Data were analysed with Oncomine expression analysis tools and Nexus Expression 2.0.Nrepresents the total number of cancer patients analysed for each cancer type. Only patients with >40% enhancement of CSN6 mRNA level compared with corresponding normal tissues were counted as ‘CSN6 overexpression’. (b) High CSN6 expression correlated with high Myc expression in pancreatic cancer. Pancreatic cancer tissue microarrays were immunostained with anti-CSN6 and anti-Myc. Micrographs of two representative pancreatic cancer specimens are shown (sale bar, 100 μm). (c) CSN6 overexpression correlated with increased levels of Myc target genes in pancreatic cancer patients and breast cancer patients. Human breast cancer patient data sets and pancreatic cancer patient data sets were retrieved from Gene Expression Omnibus (GSE1542, GSE 5847 and GSE2109) and analysed by gene set enrichment (MIT). Oncomine analysis tools and the GSEA program were used to analyse the impact of CSN6 on Myc target gene expression. (d) Enrichment score graphs showed a strong positive enrichment of Myc target gene expression in patients with CSN6-overexpressing pancreatic or breast cancer as described inc. Representative Myc target genes are shown on graphs. Black arrows indicated the position of the corresponding genes on the gene list.Pvalues calculated by the Kolmogorov–Smirnov test and false discovery rates (FDR) are shown below. Abbreviations of genes are given inSupplementary Information. (e) The model shows the CSN6’s positive effect on the expression of representative Myc target genes in human cancers. Figure 7: CSN6 is overexpressed in many cancer types and correlated with upregulation of Myc target genes. ( a ) Transcriptomic analysis revealed frequent CSN6 overexpression in human patients with cancer. Human cancer patient data sets were obtained from the Oncomine database and Gene Expression Omnibus. Data were analysed with Oncomine expression analysis tools and Nexus Expression 2.0. N represents the total number of cancer patients analysed for each cancer type. Only patients with >40% enhancement of CSN6 mRNA level compared with corresponding normal tissues were counted as ‘CSN6 overexpression’. ( b ) High CSN6 expression correlated with high Myc expression in pancreatic cancer. Pancreatic cancer tissue microarrays were immunostained with anti-CSN6 and anti-Myc. Micrographs of two representative pancreatic cancer specimens are shown (sale bar, 100 μm). ( c ) CSN6 overexpression correlated with increased levels of Myc target genes in pancreatic cancer patients and breast cancer patients. Human breast cancer patient data sets and pancreatic cancer patient data sets were retrieved from Gene Expression Omnibus (GSE1542, GSE 5847 and GSE2109) and analysed by gene set enrichment (MIT). Oncomine analysis tools and the GSEA program were used to analyse the impact of CSN6 on Myc target gene expression. ( d ) Enrichment score graphs showed a strong positive enrichment of Myc target gene expression in patients with CSN6-overexpressing pancreatic or breast cancer as described in c . Representative Myc target genes are shown on graphs. Black arrows indicated the position of the corresponding genes on the gene list. P values calculated by the Kolmogorov–Smirnov test and false discovery rates (FDR) are shown below. Abbreviations of genes are given in Supplementary Information . ( e ) The model shows the CSN6’s positive effect on the expression of representative Myc target genes in human cancers. Full size image We also analysed CSN6 gene expression in other independent patient cohorts of several types of cancer. We defined enhancement of CSN6 mRNA in tumour by >40% compared with normal tissues as ‘CSN6 overexpressing.’ We then asked whether the overexpression of CSN6 in these patients was correlated with high expression of Myc target genes. We scored 237 Myc target genes and found a positive correlation between CSN6 overexpression and elevated expression of the Myc target genes in pancreatic cancer and breast cancer patients, as evidenced by heat maps ( Fig. 7c ). Gene set enrichment score graphs clearly demonstrated that the majority of Myc target genes were upregulated in samples expressing a high level of CSN6 from both pancreatic and breast cancer patients ( Fig. 7d ). Representative Myc target genes are indicated on the graphs. These data show that the association between CSN6 and Myc is present in many types of human cancer, suggesting that the positive regulation of Myc by CSN6 may be a clinically relevant regulatory pathway in human cancers ( Fig. 7e ). In vitro studies have demonstrated that purified CSN inhibits CRL activity through its deneddylation of Cullin [53] , [54] . Importantly, CSN is in an inactive form until it binds to its substrate, CRL [55] . On the other hand, CRL is activated when it disassociates from CSN [56] . Cullin neddylation is critical for CRL activity [22] . However, these biochemical studies contradict genetic observations that the CSN is required for CRL-mediated substrate degradation, binding CRLs and facilitating their activity in vivo [23] , [57] . These observations present a paradox: if CSN5 causes Cullin deneddylation via its metalloprotease activity, why does CSN promote CRL activity? Is there another layer of regulation other than CSN5 controlling Cullin neddylation? Sequence alignment between CSN5 and CSN6 shows that CSN6 has an MPN domain, but not a JAMM motif. Thus, it raises the question of whether CSN6 can regulate Cullin neddylation. Structurally, CSN6 and CSN5 form a heterodimer through the MPN domain and the dimer is topologically knotted to engage in Cullin deneddylation [55] . Our data argue that CSN6 has a positive impact on Cullin neddylation via its competition with CSN5 for Cullin binding through its MPN domain. In the competition experiment, more CSN6 may lead to reduced CSN6–CSN5 hetreodimer, thereby affecting Cullin deneddylation [55] . Competition studies provide important insights into the role of CSN6 in maintaining Cullin neddylation and unravel, at least in part, the paradox regarding promotion of CRL activity by the COP9 complex. Replacement of some conserved residues on the MPN domain compromised CSN6’s capacity for increasing Cullin neddylation, suggesting that these residues are involved in regulation of Cullin neddylation. Furthermore, exposure to a CSN6–CSN5 chimeric protein that fused the CSN5 N-terminal domain containing the MPN motif to the CSN6 C-terminal domain did not enhance Cullin neddylation, showing that the intrinsic character of the CSN6 MPN domain is important for enhancing Cullin neddylation. Together, these results demonstrate a functional activity of the CSN6 MPN domain—engagement in facilitating Cullin neddylation. The structural studies of the CSN indicated that many different subcomplexes may exist [58] . Gusmaroli et al . [59] also showed that both CSN5 and CSN6 were present in fractions (subcomplexes) other than the CSN holocomplex. The CSN holocomplex has a tendency to dissociate to form smaller complexes. Our gel-filtration studies indicate that CSN5 and CSN6 are indeed present in different CSN subcomplexes at different CSN5/CSN6 ratios. In a side-by-side comparison of fractions of Csn6 +/− and Csn6 +/+ mouse spleen cell extracts, we observed high CSN5/CSN6 ratios in fractions of Csn6 +/− cell extracts, which in turn led to increased amounts of non-neddylated Cullin. Thus, Cullin’s binding to various CSN complexes and subsequent neddylation can be determined by the CSN5/CSN6 ratio, which may be a mechanism for dynamic regulation of Cullin neddylation. Our results indicate that CSN6 functions as part of a cycle with Cullin, CSN5 and Fbxw7, resulting in positive regulation of the Myc protein. CSN6’s association with Fbxw7 facilitates its degradation. The steady-state level of Fbxw7 protein is important in determining the ubiquitin ligase activity of the whole SCF Fbxw7 . CRL substrate adaptors, such as F-box proteins, tend to undergo autocatalytic degradation in vivo [54] , [60] . Thus, keeping the F-box stable will have an impact on the CRL, facilitating degradation of CRL targets. Importantly, we show that loss of CSN5 causes a decrease in Fbxw7. In contrast, our studies show that loss of CSN6 leads to an increase in Fbxw7. These observations imply that these two subunits function differently. Cullin neddylation decreases the steady-state expression levels of F-box proteins [60] . Here, we demonstrate that the Cullin neddylation status is controlled by CSN5 and CSN6 ratio, and that CSN6 actually preserves neddylation of Cullins, thereby increasing the autocatalytic degradation of Fbxw7. Thus our study has provided a novel mechanistic answer to how CSN6 can destabilize Fbxw7 and subsequently increase the stability of Myc. Loss of one CSN6 allele can decelerate Myc-driven lymphoma development in Eμ- Myc mice and prolong their survival. Tumour sample analysis indicates that expression of many Myc target genes was also reverted in these Eμ- Myc/Csn6 +/− mice. These studies recapitulate the positive relationship between CSN6 and Myc in vivo . Noticeably, reduced expression of Csn6 in Eμ- Myc background can also contribute to p53 stabilization in 33% of Eμ- Myc/Csn6 +/− lymphomas when compared with Eμ- Myc/Csn6 +/+ , suggesting that both CSN6-mediated p53 downregulation and CSN6-mediated Myc elevation contribute to lymphomagenesis of this system ( Fig. 6 ). CSN6 is an oncogene frequently overexpressed in breast cancer. We further found here that CSN6 gene overexpression is quite common in many types of cancer. Significantly, CSN6 overexpression positively correlates with Myc protein expression and the gene expression signature of Myc target genes in human breast and pancreatic cancer samples. Therefore, our study demonstrated that CSN6 overexpression can account for Myc overexpression in some of the cancers and provided important insights into the mechanism of Myc overexpression in cancers. The observation that CSN6 acts as a positive regulator of Myc raises the possibility that inhibiting the CSN6 signalling axis may be an efficient therapeutic approach in Myc-overexpressing cancers. Cell transfection and shRNA-mediated silencing Human U2OS and 293T cells (obtained from ATCC) were cultured in Dulbecco's modified Eagle's medium/F12 medium supplemented with 10% fetal bovine serum. HCT116 and HCT116 Fbxw7 −/− cells were kindly provided by Dr Bert Vogelstein and cultured in McCoy’s 5A medium supplemented with 10% fetal bovine serum. For transient transfection, MEFs, 293T, U2OS and HCT116 cells were transfected with plasmids using Lipofectamine TM 2000 (Invitrogen). For the lentivirus infection system, 293T cells were cotransfected with CSN5, CSN6 or Luciferase shRNA (as control) along with the packaging plasmid (ΔVPR8.9) and envelope plasmid (VSV-g) using Lipofectamine 2000 reagents according to the manufacturer’s instructions. MEFs, HCT116 and U2OS cells were infected with the lentivirus particles containing CSN5, CSN6 or Luciferase control shRNA. CSN6 shRNA plasmid (#1:NM_006833.4-1084s1c1, #2: NM_006833.4-165s1c1), CSN5 shRNA plasmid (NM_006833.4-1084s1c1) and Luciferase shRNA Control Vector (SHC007) were purchased from Sigma-Aldrich and had these target sequences: CSN6 shRNA #1: 5′-CCGGCTTGAGAGAAACCGCTGTCATCTCGAGATGACAGCGGTTTCTCTC AAGTTTTTG -3′ CSN6 shRNA #2: 5′-CCGGCCCTTGTCATTCTCAACATCTCTCGAGAGATGTTGAGAATGAC AAGGGTTTTTG -3′ CSN5 shRNA: 5′-CCGGCGTGGAAGAGAAGATTATCATCTCGAGATGATAATCTTCTCTTCC ACGTTTTTG -3′ Luciferase shRNA: 5′-CCGGCGCTGAGTACTTCGAAATGTCCTCGAGGACATTTCGAAGTACT CAGCGTTTTT -3′ For knocking down CSN6 in 293T cells, pSilencer 1.0-U6 plasmid containing Csn6 shRNA oligos (sequence: 5′-ACGTGCAACACAATGAACCTTCAAGAGAGTTCATTGTGTTGCACGTTTT TTTCCGGTGCACGTTGTGTTACTTGGAAGTTCTCTCAAGTAACACAACGTGCAAAAAAATTAA-3′) were cotransfected with indicated plasmids. Small interfering RNAs (siRNAs) for Cullin-1 (ON-TARGETplus SMARTpool siRNA L-004086-00-0005) and siRNA control (ON-TARGETplus Non-targeting Pool), were purchased from Thermo Scientific Dharmacon. Plasmids and reagents The PCR-generated DNA fragment of the human Csn6 gene was subcloned into pCMV5 to generate a construct that encodes CSN6 with a Flag-tagged sequence or a green fluorescent protein (GFP)-tagged sequence, or into pCDNA6 to encode a Myc-tagged sequence. Mutant pcDNA6-Myc-CSN6-MPN-GVGG, pcDNA6-Myc-CSN6-MPN-KQV and pcDNA6-Myc-CSN6-MPN-GWY constructs were generated by using a site-directed mutagenesis kit (Stratagene) according to the manufacturer’s instructions. Plasmids for Fbxw7α, Fbxw7β, Fbxw7γ and its ΔF mutants were described previously [35] . Fbxw7α ΔD (D domain, 230aa–280aa deletion), Fbxw7α N (1aa–360aa) and Fbxw7α WD40 (361aa–707aa) mutants were generated in Flag-tagged pCMV5 vector. Skp2 −/− MEF cells and His-ubiqutin wt, His-ubiqutin-K48R and His-ubiqutin-K63R plasmids were kindly provided by Dr Hui-Kuan Lin (Department of Molecular and Cellular Oncology, MD Anderson Cancer Center). Nedd8 plasmid was kindly provided by Dr Edward T. H. Yeh (Department of Cardiology, MD Anderson Cancer Center). Dominant-negative Ubc12-HA (dn-Ubc12-HA) plasmid was kindly provided by Dr Thilo Hagen (Department of Biochemistry, Yong Loo Lin School of Medicine, National University of Singapore). Fluorescein isothiocyanate (FITC) Annexin V Apoptosis Detection kit was purchased from BD Pharmingen. MG132, cycloheximide and puromycin were purchased from Sigma. Mouse models Csn6 +/− mice bear one null allele, which was disrupted by insertional mutagenesis into the ninth intron of the Csn6 gene. These mice are born at mendelian ratios and are viable into adulthood and fertile without any manifest phenotype. The homozygous Csn6 −/− phenotype is embryonically lethal. The CSN6 knockout and PCR-based genotyping strategies are described elsewhere [15] . The PCR primers for Csn6 +/− mice were as follows: forward, 5′-GCATCGAGCTGGGTAATAAGCGTT GGCAAT -3′; reverse, 5′-GACACCAGACCAACTGGTAATGGTAGCGAC -3′. Eμ- Myc transgenic mice were maintained and studied in a heterozygous background. Mice were monitored twice a week for signs of morbidity and tumour development. Tumours in peripheral lymph nodes were monitored by palpation. Sick mice were killed, and tumours and lymphoid organs were subjected to histologic analysis or processed for further analysis. The PCR primers for Eμ- Myc transgenic mice were as follows: forward, 5′- GGTTTAATGAATTTGAAGTTGCCA -3′; reverse, 5′- TTCTTGCCCTGCGTATATCAGTC -3′. All protocols involving the use of animals were approved by the IACUC committee at MD Anderson Cancer Center. Preparation of MEFs and flow cytometry for B cell apoptosis MEF cells were prepared from 13.5-day embryos derived from Csn6 +/+ and Csn6 +/− mice. Head, tail and viscera were removed, and the remaining body was minced and dispersed in 0.25% trypsin/EDTA and incubated in 5% CO 2 at 37 °C for 30 min. The large fragments were removed, and the remaining cell suspension was plated in 100-mm plates and incubated at 37 °C until confluent. We obtained single-cell suspensions by pressing the spleen through nylon cell strainers or by crushing the leg bones of euthanized 4-week-old mice and subsequent hypotonic lysis of red blood cells (eBioscience). To isolate B cells, we incubated single-cell suspensions from spleen or bone marrow with B220 MicroBeads (Miltenyi Biotech) and enriched them by magnetic cell sorting according to the manufacturer’s instructions (Miltenyi Biotech). Primary bone marrow-derived B cells were cultured in RPMI 1640 medium supplemented with 10% fetal calf serum with recombinant murine interleukin-7 (50 ng ml −1 ) (PeproTech Inc.). The isolated B cells were treated with cycloheximide for the indicated durations for turnover assays. Apoptosis of B cells was determined by two-colour analysis using propidium iodide (PI) and FITC-conjugated annexin V according to the manufacturer’s instructions. After isolation of B cells from mouse spleens, the B cells were stained with PI and annexin V-FITC and then analysed using a FACScan flow cytometer (BD Biosciences Pharmingen) with a Macintosh G5 workstation (Apple Computer). Ubiquitination assays For in vivo ubiquitination assays, 293T cells were cotransfected with the indicated plasmids. Nickel-nitrilotriacetic acid (Ni-NTA) agarose was used to pull down ubiquitinated c-Myc or Fbxw7 proteins. After 48 h of transfection, cells were treated with 50 μg ml −1 MG132 for 6 h and subjected to lysis in phosphate-buffered saline (PBS) solution containing 1% Nonidet P-40 and 10 mM imidazole. Ni-NTA-agarose beads (Qiagen, Inc.) were then added to cell extracts (1,500 μg) and the mixtures rotated at room temperature for 4 h. Precipitates were washed three times with PBS containing 1% Nonidet P-40 and 20 mM imidazole and boiled in SDS-polyacrylamide gel electrophoresis sample buffer. Protein complexes were then separated on 8% SDS-polyacrylamide gels and probed with anti-HA antibody to reveal ubiquitinated c-Myc or probed with anti-Flag antibody to observe ubiquitinated Fbxw7. For detection of ubiquitinated protein in vitro , proteins were incubated with different combinations of ubiquitin (200 pmol), E1 (2 pmol), E2-UbcH5a/5b (10 pmol), in vitro translated 35 S-labelled proteins and ATP (2 mM) in a total volume of 50 μl for 1 h at 37 °C. Reaction products were detected by X-ray film exposure. Turnover assay The cells were transfected with indicated plasmids. Cycloheximide was added into the media at 60 μg ml −1 of final concentration. The cells were harvested at the indicated time points after CHX treatment. The protein levels were analysed by immunoblotting. In other case, the cells were pulse-labelled with 35 S- methionine, and the interested protein was immunoprecipitated from indicated cell lysates. The density of protein was measured by densitometer and the integrated optical density was measured. Neddylation assay For the in vivo neddylation assays, 293T cells were cotransfected with His-tagged Cullin-1 and indicated plasmids. Ni-NTA agarose was used to pull down Cullin-1 proteins. After 48 h of transfection, cells were subjected to lysis in PBS containing 1% Nonidet P-40 and 10 mM imidazole. Ni-NTA-agarose beads were added to cell extracts (1,500 μg) and the mixtures rotated at room temperature for 4 h. Precipitates were washed three times with PBS containing 1% Nonidet P-40 and 20 mM imidazole and then boiled in SDS-polyacrylamide gel electrophoresis sample buffer. Protein complexes were then separated on 8% SDS-polyacrylamide gels and probed with anti-Nedd8 antibody (Enzo Llife Ssciencess, PW9340) to reveal neddylated Cullin-1. BrdU incorporation assay For assay of BrdU incorporation into B cells, animals were injected intraperitoneally with 0.04 μg kg −1 BrdU in sterile PBS; the animals were killed 12 h later and their spleens isolated. Splenic B cells (10 × 10 6 ) were suspended and treated with 2N HCl/Triton X-100 for 1 h at 37 °C to expose incorporated BrdU. This was followed by incubation with FITC-conjugated anti-BrdU-antibody (PharMingen, 33284X). Total DNA content was stained with PI. Flow cytometry was performed on a FACScan flow cytometer. Data were analysed with Cellquest graphics software (Becton Dickinson). Quantitative RT–PCR Total RNA was extracted with the use of TRIZOL reagent (Invitrogen) according to the manufacturer’s instructions. Reverse transcription was performed by using SuperScript III First-Strand kit (Invitrogen). Each cDNA sample (10 ng) was amplified in triplicate with iQ SYBR Green Supermix PCR kit (Bio-Rad) for 40 cycles on a Bio-Rad system (iCycler Thermal Cycler). Sequences for primers are shown in Supplementary Table 2 . Fold gene amplifications for multiple genes were analysed and visualized with Cluster and TreeView software (Eisen, MB), and the results are presented in the form of heat maps. Immunoblot and immunohistochemistry Cells were harvested and subjected to lysis with lysis buffer (50 mM Tris-HCl pH 7.5, 0.15 M NaCl, 1% NP-40 and 1 mM EDTA), Complete Protease Inhibitor Cocktail (Roche Applied Science), 1 mM PMSF, 1 mM NaF and 1 mM sodium orthovanadate; they then were subjected to sonication. Lysates were immunoprecipitated with indicated antibodies. The following antibodies were used for immunoblot analysis: CSN6 (BIOMOL international, PW8295), CSN5 (GeneTex, JAB1, GTX70207), CSN7 (BIOMOL international, PW8300), CSN8 (BIOMOL international, PW8290), Skp1 (BD Transduction Laboratories, 610530), Skp2 (Invitrogen, 32-3300), Cullin-1 (Invitrogen, 71-8700), Cul-4A (Proteintech Group, 14851-1AP), Nedd8 (Enzo Life Sciences, PW9340), c-Myc (Santa Cruz Biotechnology, 9E10, sc-40), Cyclin E (Santa Cruz Biotechnology, sc-481), c-Jun (Cell Signaling Technology, 9162), Cdk4 (Santa Cruz Biotechnology, sc-601), p21Cip1 (Santa Cruz Biotechnology, F-5, sc-6246), p27Kip1 (BD Transduction Laboratories, 610241 ), p53 (Santa Cruz Biotechnology, FL-393, sc-6243), Fbxw7 (Invitrogen, 39-5800), Max (Santa Cruz Biotechnology, C-17, sc-197), Ubiquitin (Zymed, 13-1600), Flag (Sigma, F3165), GFP (Santa Cruz Biotechnology, sc-9996), HA (Roche, 11666606001), Tubulin (Sigma, T-5168) and Actin (Sigma, A2066). Original films of immunoblotting were in Supplementary Figs 9–15 . For immunohistochemical analysis, tissues were fixed in 10% formalin and embedded in paraffin in accordance with standard procedures. Sections were stained with anti-Fbxw7 and anti-CSN6 antibodies. Diaminobenzidine was used as a chromogen, and haematoxylin was used for counterstaining. Pathologic analysis IHC was performed on a tissue microarray consisting of primary pancreatic tumour specimens from 123 patients (IRB protocol number is LAB05-0854) who underwent initial pancreatico-duodenectomy at UTMDACC between 1990 and 2004. Informed consent was obtained as approved by IRB. Immunohistochemical staining for CSN6 and Myc was performed on 5-μm unstained sections from the tissue microarray blocks. Sections were incubated for 90 min at 37 °C with primary antibodies against CSN6 or Myc at a 1:100 dilution. The sections were subjected to standard avidin-biotin immunohistochemical analysis (Vector Laboratories). The staining results were evaluated by a board-certified pathologist (H.W.). Statistical analysis Differences in proportions of Eμ- Myc lymphomas expressing various proteins were analysed by the Fisher exact test. Other normally distributed quantitative parameters between two groups were compared with the Student’s t -test, and those among >2 groups with one-way analysis of variance, with post hoc intergroup comparison using the Tukey test. Kaplan–Meier survival curves were compared between two groups using the log-rank test. How to cite this article: Chen, J. et al . CSN6 drives carcinogenesis by positively regulating Myc stability. Nat. Commun. 5:5384 doi: 10.1038/ncomms6384 (2014).